Predictive modelling-based design and experiments for synthesis and spinning of bioinspired silk fibres Scalable computational modelling tools are required to guide the rational design of complex hierarchical materials with predictable functions. Here, we utilize mesoscopic modelling, integrated with genetic block copolymer synthesis and bioinspired spinning process, to demonstrate de novo materials design that incorporates chemistry, processing and material characterization. We find that intermediate hydrophobic/hydrophilic block ratios observed in natural spider silks and longer chain lengths lead to outstanding silk fibre formation. This design by nature is based on the optimal combination of protein solubility, self-assembled aggregate size and polymer network topology. The original homogeneous network structure becomes heterogeneous after spinning, enhancing the anisotropic network connectivity along the shear flow direction. Extending beyond the classical polymer theory, with insights from the percolation network model, we illustrate the direct proportionality between network conductance and fibre Young's modulus. This integrated approach provides a general path towards de novo functional network materials with enhanced mechanical properties and beyond (optical, electrical or thermal) as we have experimentally verified. Natural protein biomaterials such as silk have been the subject of intensive research due to the extraordinary properties with versatile potential applications [1] , [2] . Among them, spider silks possess exceptional mechanical properties with toughness comparable to Kevlar [3] and strength comparable to steel, yet by weight is six times lighter [4] . Silks, due to biocompatibility [5] and biodegradability [6] , are useful protein-based materials for biomedical applications such as wound sutures [7] , artificial nerve guides [8] , tissue regeneration [9] , [10] and gene [11] or drug delivery [12] . Despite the simple amino acid building blocks for silk proteins, spiders and silkworms produce silks with remarkable mechanical and adhesive properties by engineering nanoscale protein aggregate morphologies via multiple stages of spinning, relying at its foundation on self-assembly and shear flow-induced focusing along their microchannel-like spinning ducts. Silk protein sequence alterations, together with fibre-processing parameters, allow for a huge design space for new polymeric materials. The molecular-level microstructure formation of polymer aggregates via self-assembly has been recognized as a very important process that determines the material properties. To fully harness these processes to generate defined material features, there have been extensive efforts [13] , [14] to artificially synthesize the silk fibre with regenerative [15] and synthetic (or recombinant) [16] , [17] , [18] silks. Using recombinant silk is also more practical and cost effective than harvesting silk materials from spider farms and, therefore, has great potential for large-scale manufacturing. Yet, the design and implementation of synthetic imitations have been hindered by incomplete knowledge about the interplay between protein structure, fibre processing and fibre properties. These limitations have resulted in an inability to fully recapitulate the suite of remarkable mechanical properties of silk. Synthetic silk protein sequences of this work contain three major building blocks named ‘A’ (poly(alanine) containing, hydrophobic domain), ‘B’ (GGX (X=R, L, Y or Q) rich, hydrophilic domain) and ‘H’ (hexahistidine fusion tag, introduced for facile purification, hydrophilic domain same as ‘B’). ‘A’ and ‘B’ represent an abstraction of the natural silk protein sequence in which hydrophobic and hydrophilic domains are arranged repetitively into a multiblock copolymer. The amino-acid sequence in each domain is also identical to the native sequence in the major ampullate spidroin (MaSp1, Accession Number: P19837.3) of Nephila clavipes [19] , [20] . 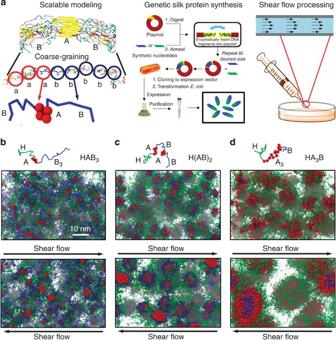Figure 1: Integrated fibre design framework and DPD simulation snapshots. (a) Illustration of the integrated framework that synergistically combines scalable modelling using coarse-graining, genetic silk protein synthesis and shear flow spinning process. Mesoscopic DPD simulation snapshots of the recombinant short silk peptides: (b) HAB3, (c) H(AB)2and (d) HA3B, with coarse-grained representations (top panel), snapshots after equilibration (middle panel) and after shear flow (bottom panel). Hydrophobic ‘a’ beads form aggregates (clusters composed of cross-linked β-crystals via hydrogen bonds) and hydrophilic ‘b’ beads form corona structures around the cluster and physical links between two clusters. The HAB3solution exhibits small micellar aggregates (<5 nm in diameter), with a minor increase in micelle size after shear. In contrast, the HA3B solution exhibits large micellar aggregates (>10 nm in diameter) with enlarged inhomogeneous globular aggregates after shear (15∼20 nm in diameter), which leads to the clogging of the spinning channel. The H(AB)2solution exhibits middle-sized homogeneous aggregates (∼5 nm in diameter) with enlarged aggregates after shear (∼10 nm in diameter). Note that water beads are not shown for clarity and the scale bar applies for all snapshots. Colour code: red beads—hydrophobic ‘a’ beads in the ‘A’ domain, blue lines—hydrophilic ‘b’ beads in the ‘B’ domain and green lines—hydrophilic ‘b’ beads in the ‘H’ domain. Specifically, the sequences ( Supplementary Table 1 ) for the ‘A’ and ‘B’ domains are GAGAAAAAGGAGTS and QGGYGGLGSQGSGRGGLGGQTS , respectively. For the ‘A’ domain, the hydrophobic alanine ( A ) amino acids are responsible for the self-assembly of proteins into aggregates via β-sheet stacking, whereas the glycine ( G ) amino acids facilitate the hydrogen bonding between β-sheets. As a result, the hydrophobic ‘A’ domains form stiff and strong β-sheet crystals, whereas the hydrophilic ‘B’ domains form disorganized and extensible amorphous regions. Theoretical models for describing the self-assembled morphologies of block copolymers are still limited to very simple copolymer structures [21] , in which Flory–Huggins parameters ( χ AB ) are used to quantify the degree of incompatibility between the hydrophobic and the hydrophilic domains. For example, the self-consistent mean-field theory can only predict phase diagrams of pure diblock or triblock copolymers in bulk or with solvents [22] , but not the molecular structures in detail [23] . On the other hand, our recent atomistic simulations revealed various structural details and mechanics of the crystalline and amorphous regions of the silk protein in aqueous environments [24] , [25] , [26] . However, the atomistic simulations are not efficient enough to study the self-assembly process of a large number of proteins or polymers in the mesoscale. Therefore, scalable computational modelling approaches are required to study more complicated protein-like multiblock copolymers, in particular, protein sequences with ∼ 20 different amino-acid building blocks in aqueous environments. With the above in mind, in this paper, we develop a coarse-grained description of silk proteins as multiblock copolymers based on the mesoscopic dissipative particle dynamics (DPD) simulation [27] , [28] (see Methods), and apply the model to reveal the critical processing conditions and design parameters that control silk fibre assembly. We also validate the model against silk protein biosynthesis and characterization, and syringe needle fibre spinning and tensile testing (see Methods). This integrated modelling and experimental framework is illustrated in Fig. 1a . We reveal the structural evolution of the silk protein solution under shear flow and study how the ‘A’–‘B’ domain ratio and the protein molecular weight (polymer chain length) affect the fibre formation process. Our simulation results and polymer network analysis suggest that intermediate ‘A’–‘B’ domain ratio leads to homogeneous and well-connected polymer solution, which is the key during the fibre-spinning process. We also reveal that, in addition to the β-sheet crystal content, longer chains are crucial for the formation of robust fibres. The shear flow further enhances the alignment of longer polymers and the size of the β-sheet crystal, which leads to gelation and fibre assembly [29] . Networks formed by shorter polymers are easily disrupted by the shear flow. To obtain a general polymer design principle, we extend beyond the classical polymer theory, which describes only homogeneous polymer aggregates before spinning with insights from the percolation network model, which also describes heterogeneous polymer networks after spinning. This molecular-level design principle for mechanically robust silk fibres is finally realized in our spinning and nanoindentation experiments. Figure 1: Integrated fibre design framework and DPD simulation snapshots. ( a ) Illustration of the integrated framework that synergistically combines scalable modelling using coarse-graining, genetic silk protein synthesis and shear flow spinning process. Mesoscopic DPD simulation snapshots of the recombinant short silk peptides: ( b ) HAB 3 , ( c ) H(AB) 2 and ( d ) HA 3 B, with coarse-grained representations (top panel), snapshots after equilibration (middle panel) and after shear flow (bottom panel). Hydrophobic ‘a’ beads form aggregates (clusters composed of cross-linked β-crystals via hydrogen bonds) and hydrophilic ‘b’ beads form corona structures around the cluster and physical links between two clusters. The HAB 3 solution exhibits small micellar aggregates (<5 nm in diameter), with a minor increase in micelle size after shear. In contrast, the HA 3 B solution exhibits large micellar aggregates (>10 nm in diameter) with enlarged inhomogeneous globular aggregates after shear (15 ∼ 20 nm in diameter), which leads to the clogging of the spinning channel. The H(AB) 2 solution exhibits middle-sized homogeneous aggregates ( ∼ 5 nm in diameter) with enlarged aggregates after shear ( ∼ 10 nm in diameter). Note that water beads are not shown for clarity and the scale bar applies for all snapshots. Colour code: red beads—hydrophobic ‘a’ beads in the ‘A’ domain, blue lines—hydrophilic ‘b’ beads in the ‘B’ domain and green lines—hydrophilic ‘b’ beads in the ‘H’ domain. Full size image Effects of domain ratio and shear flow To examine the effect of hydrophobic–hydrophilic (‘A’–‘B’) domain ratios on fibre formation, three simple short peptide sequences with similar polymer chain length (molecular weight) are considered: HA 3 B, H(AB) 2 and HAB 3 ( Fig. 1b–d ), with different domain ratios 3:1, 1:1 and 1:3, respectively. The ‘A’ domain is modelled using five hydrophobic ‘a’ beads and the ‘B’ domain is modelled using seven hydrophilic ‘b’ beads. DPD simulation results on the aqueous solutions of HAB 3 , H(AB) 2 and HA 3 B right after equilibration (before shear flow) is shown in Fig. 1b–d , middle panel. We expect that the electrostatic interactions between silk proteins will be relatively weak here, because the degree of protonation or de-protonation is quite low due to the use of organic solvents rather than water. Therefore, electrostatic interactions are currently neglected in the DPD model and such effect will be considered in future studies to better mimic the ionic aqueous environment in the natural spider silk-spinning process [30] , in which the silk protein should be modelled as a polyelectrolyte. Starting with randomized polymer solutions, the equilibration of the system results in the formation of spherical polymer micelle structures in which hydrophobic ‘a’ beads in the ‘A’ domain aggregate (or cross-linked via hydrogen bonding) into multiple crystalline clusters (β-sheet crystals) surrounded by the corona composed of hydrophilic ‘b’ beads extended towards the aqueous environment. The size of the micelles increases as the ‘A’–‘B’ domain ratio increases and follows the trend: HA 3 B>H(AB) 2 >HAB 3 , due to stronger hydrophobic attractions among the larger amounts of ‘a’ beads. This computational observation is in good agreement with scanning electron microscopy (SEM) images comparing the three sequences synthesized and purified, as well as the Fourier transform infrared (FTIR) spectroscopy measurements that provide the percentages of protein secondary-structure contents (see Supplementary Methods and Supplementary Fig. 3 ). The observed trend that block copolymers with larger hydrophobic–hydrophilic domain ratios form larger aggregates is in good agreement with other theoretical [31] and experimental [21] studies on self-assembly of block copolymers or in general, amphiphilic molecules in aqueous solutions. Under shear flow, polymer chains extend along the flow stream and the size of micelles increases by merging multiple micelles as the ‘a’ beads cluster further together ( Fig. 1b–d , bottom), in good agreement with earlier theoretical studies on block copolymer micelles, which elongate and aggregate under shear flow [32] . The aggregate elongation or spherical-to-cylindrical transition under shear flow is not significant for the short sequences studied here, including HAB 3 , H(AB) 2 and HA 3 B. Such transition is more obvious for longer sequences (discussed later). The change of micelle size in the HAB 3 solution after shearing is modest because each micelle is surrounded by a dense corona of longer hydrophilic chains ( Fig. 1b , bottom). In contrast, in the case of the HA 3 B solution, the micelles are lumped into globular structures owing to their larger hydrophobic cores and less steric repulsion from the smaller hydrophilic corona ( Fig. 1d , bottom). These simulation results are consistent with previous experiments [33] , [34] in which pure solutions of the HAB 3 sequence did not form fibres and the HA 3 B solution suffered from clogging during the microfluidic processing. Finally, in the case of H(AB) 2 , the flow shearing process results in a homogeneous solution of micelles with the size doubled ( Fig. 1c , bottom). Polymer clusters composed of the ‘A’ domain exhibit physical connections between them when they share the amorphous ‘B’ domains of the same polymer, which is the key prerequisite for them to assemble into robust silk fibres. To effectively visualize the connectivity between the clusters composed of the particles that define the ‘A’ domains, we devised a novel node–bridge network diagram (see Methods) in which a ‘node’ represents the centre of mass of the cluster and a ‘bridge’ represents the physical link between two nodes. Here, the thickness of each bridge is linearly proportional to the multiplicity of the connections, that is, the number of polymer chains through which two nodes connect. The node–bridge diagrams in Fig. 2a show that only the H(AB) 2 sequence enables weak but connected polymer networks both before and after shear flow, compared with the HAB 3 and HA 3 B sequences. Time evolution of the network properties ( Fig. 2b ) show that the median number of ‘a’ beads per node (as a measure of the aggregate size) is larger for higher ‘A’–‘B’ domain ratios, and that the aggregate size increases significantly after shear flow due to flow-focused concentration. Note that the median value is used instead of the mean value because the cluster size distribution could be highly skewed. In addition, the total number of bridges formed remains zero for high and low ‘A’–‘B’ domain ratios ( Fig. 2c ), which suggests the advantage of the intermediate domain ratio to allow connected polymer networks and its potential for fibre formation. 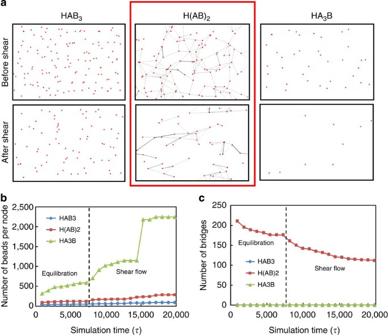Figure 2: Polymer network structures for the HAB3, H(AB)2and HA3B sequences. (a) Polymer network analysis leads to the node–bridge diagram of the three peptide sequences before and after shear flow (all correspond to the simulation snapshots inFig. 1). Only the H(AB)2sequence exhibit weak network connectivity, whereas the other two sequences do not form any network. Time evolution of the simulated polymer network properties during equilibration and shear flow: (b) median number of ‘a’ beads per node as a measure of the aggregate size and (c) the total number of bridges as a measure of the connectivity. The median size of each aggregate or cluster (b) is increased during the shear flow and the trend is consistent withFig. 1, while the total number of bridges (c) is reduced for H(AB)2during the shear flow and remains zero for both HAB3and HA3B. These results clearly show the advantage of the H(AB)2sequence with the intermediate ‘A’–‘B’ domain ratio to form connected polymer networks (highlighted by the red rectangle). Figure 2: Polymer network structures for the HAB 3 , H(AB) 2 and HA 3 B sequences. ( a ) Polymer network analysis leads to the node–bridge diagram of the three peptide sequences before and after shear flow (all correspond to the simulation snapshots in Fig. 1 ). Only the H(AB) 2 sequence exhibit weak network connectivity, whereas the other two sequences do not form any network. Time evolution of the simulated polymer network properties during equilibration and shear flow: ( b ) median number of ‘a’ beads per node as a measure of the aggregate size and ( c ) the total number of bridges as a measure of the connectivity. The median size of each aggregate or cluster ( b ) is increased during the shear flow and the trend is consistent with Fig. 1 , while the total number of bridges ( c ) is reduced for H(AB) 2 during the shear flow and remains zero for both HAB 3 and HA 3 B. These results clearly show the advantage of the H(AB) 2 sequence with the intermediate ‘A’–‘B’ domain ratio to form connected polymer networks (highlighted by the red rectangle). Full size image The above findings suggest that the delicate balance between the ‘A’ and ‘B’ domains are critical for the polymer network connectivity: for large ‘A’–‘B’ domain ratios, there are not enough ‘B’ domains to form the bridges, whereas for small ‘A’–‘B’ domain ratios, the cluster is too small and fragile to maintain the bridges between them. Therefore, the intermediate ‘A’–‘B’ domain ratio examined here (1:1 for H(AB) 2 ) provides the optimal combination of robust cluster formation and network connectivity. Interestingly, this optimal 1:1 ratio matches the hydrophobic/hydrophilic domain ratio in the native MaSp1 sequence of Nephila clavipes [19] , [22] , suggesting an evolutionary principle to adapt certain material properties. For different spider species that already possess close-to-optimal domain ratios, previous literature implies that the major ampullate (dragline) silk mechanical properties could be greatly affected by the small difference in the alanine fractions (one of the major building blocks of the ‘A’ domain here) of the corresponding silk proteins [35] . For example, the alanine fraction of Nephila clavipes dragline silk is 21.1 ∼ 27.5%, higher than the alanine fraction of 17.6% for the Araneus diadematus dragline silk, which could lead to the higher Young's modulus of the former silk (8 ∼ 14 GPa) compared with the latter one ( ∼ 4 GPa, ref. 35 ). Therefore, the polymer domain ratio here also has a strong influence on the structure and mechanics of silk from different spider species. A positive correlation may exist between the alanine fractions in the silk protein and the Young's modulus of silk materials. Other mechanical properties, such as ultimate tensile strength/strain and toughness, will depend on additional factors of the protein sequence, including the amorphous structure of the protein and the resulting protein extensibility. Effects of sequence length and shear flow Inspired by the fact that long chain, high molecular weight regenerative silk fibroins have been used as a good additive to fabricate silk fibres [34] , we then pursued new design improvements using much longer protein sequences based on the model-predicted H(AB) 2 sequence with the optimal ‘A’–‘B’ domain ratio. Towards this effort, we carried out a set of new simulations on the H(AB) n ( n =2, 4, 8 and 12) sequences with increasing multiblock copolymer chain length as the number of repeated units n increases ( Fig. 3a,b ). The molecular weights of different sequences also range from 11,654 to 43,731 Da for n =2 to 12. In comparison, various MaSp sequences have been shown to contain short peptide motifs that are repeated multiple times with various combinations to form repetitive structural modules, which range in size for the core sequence from n =19 to 46 (ref. 36 ). For example, the native MaSp1 sequence possesses short peptide motifs (accession number: P19837.3) with n =20 (refs 19 , 22 ). The messenger RNA sizes for MaSp1 and MaSp2 were shown to be ∼ 12.5 and 10.5 kb, respectively, generating proteins around 350 kDa that contains also the carboxy (C)-/amino (N)-terminals and the spacer groups [22] . Although the simulations and experiments here focus on shorter peptides with n ≤12 as a proof of concept, they represent the major structural modules of native silk proteins for self-assembly and the findings here should hold their generality. We are also in the progress of expressing and synthesizing longer recombinant silk proteins with n values from 20 to 100. 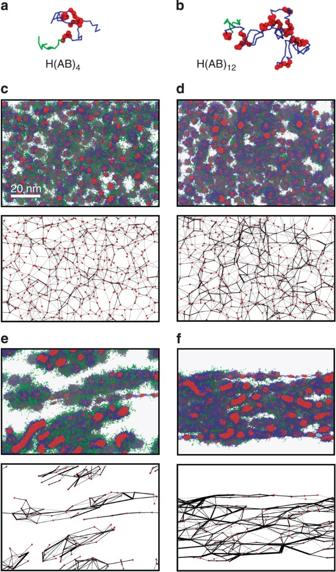Figure 3: DPD simulation snapshots and polymer network structures for the H(AB)nsequences. (a,b) Single protein snapshots for H(AB)4and H(AB)12. (c,d) H(AB)4and H(AB)12results before shear flow (after equilibration). (e–f) H(AB)4and H(AB)12results after shear flow. Below each simulation snapshot, the corresponding node–bridge diagram is plotted where hydrophobic crystals are represented as red nodes and physical bridges as black lines. The thickness of the black lines is linearly proportional to the multiplicity of the bridge (number of connections). Colour code is the same as inFig. 1. Note that water beads are not shown for clarity and the scale bar applies for all the snapshots. Figure 3: DPD simulation snapshots and polymer network structures for the H(AB) n sequences. ( a , b ) Single protein snapshots for H(AB) 4 and H(AB) 12 . ( c , d ) H(AB) 4 and H(AB) 12 results before shear flow (after equilibration). ( e – f ) H(AB) 4 and H(AB) 12 results after shear flow. Below each simulation snapshot, the corresponding node–bridge diagram is plotted where hydrophobic crystals are represented as red nodes and physical bridges as black lines. The thickness of the black lines is linearly proportional to the multiplicity of the bridge (number of connections). Colour code is the same as in Fig. 1 . Note that water beads are not shown for clarity and the scale bar applies for all the snapshots. Full size image The simulated equilibrium structures of the different H(AB) n sequences exhibit homogeneously distributed clusters of similar but slightly increased sizes for longer chains ( Fig. 3c,d ) for comparisons between n =4 and 12). This finding is consistent with experimental atomic force microscopic (AFM) images of the protein solution (see Supplementary Methods and Supplementary Fig. 4a ). However, the network node–bridge diagram of longer chains shows more densely distributed bridges and greatly enhanced the total number of bridges compared with shorter ones ( Fig. 3c,d , bottom). Furthermore, for longer chains, we find more multi-connected bridges (thicker black lines in the diagram). The different sequences also show distinct configuration change after the shear flow ( Fig. 3e,f for comparison between n =4 and 12). Aggregate elongation or spherical-to-cylindrical transition under shear flow is very significant for the longer sequences here ( n ≥4), consistent with previous simulation results [32] . As the polymer chains stretch along the fibre axis ( x axis) under shear flow, the cross-linked β-sheet crystals (composed of the ‘A’ domains) grow in size until it reaches the steady state for which the overall crystal size increases significantly. This is also consistent with experimental FTIR-derived percentages of protein secondary-structure contents for the protein aggregates (see Supplementary Methods and Supplementary Fig. 4b ), in which the β-sheet content increases by threefold after fibre spinning. Interestingly, from node–bridge diagrams, we find that the number of multi-connected bridges is greatly enhanced after shear flow, but only longer sequences exhibit homogeneous and continuous networks along the x axis while shorter sequences exhibit only isolated and discontinuous networks ( Fig. 3e,f , bottom). Our simulation well explains, for the first time at the molecular level, the previously observed monotonic increasing trend in fibre mechanics as the recombinant silk protein chain becomes longer, even up to 96 repeated units (molecular weight=285 kDa) without plateau [37] . Time evolutions of the polymer network properties ( Fig. 4a,b ) confirm the observed changes of the median cluster size and total number of bridges of the H(AB) n sequences during shear flow and subsequent mechanical tensile testing. As discussed earlier, the cluster size shows a weak dependence on the peptide length because it is determined primarily by the composition of the hydrophobic ‘A’ domains, although shear flow can greatly enlarge the cluster size. The total number of bridges shows a significant dependence on the polymer chain length, however, the total number of bridges is not enhanced at all during shear flow, which is probably due to the flow-induced perturbation and disruption of the network in all directions (isotropic). In analogy to the percolation network, we also computed the distribution of the number of connected nodes for H(AB) 4 and H(AB) 12 sequences ( Fig. 4d ). Two nodes with only single connection between them can be considered as dangling bonds, which do not contribute to the materials strength because they are not stretched under tension. The fraction of such wasted connection is zero for the longer H(AB) 12 sequence, suggesting the advantage of longer chain length in spinning robust silk fibres. 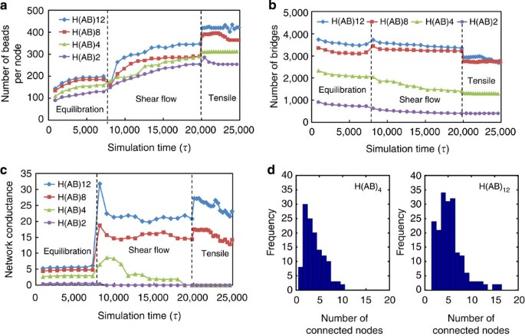Figure 4: Time evolution of the polymer network properties for the H(AB)nsequences. (a) Median number of ‘a’ beads per node as a measure of the aggregate size. (b) The total number of bridges as a measure of the connectivity. (c) The polymer network conductance as a measure of the degree of protein alignment. During both equilibration and shear flow, the median sizes of nodes do not vary a lot among all sequences (a), but longer copolymers have significantly more bridges (b). During shear flow, copolymers are stretched under shear flow and the cross-links are continuously broken and reformed until the steady state is reached for the simulated polymer properties ina–c. Although the network connectivity is not increased (in fact, it drops by a little due to shearing-induced perturbation) during shear flow (b), the network conductance for the long sequences (n=8 and 12) are greatly enhanced due to the shearing-induced polymer alignment (c). The discontinuity between shear flow and tensile stretching periods ina–cis due to the stress relaxation simulation (results not reported here) in between the two periods. Interestingly, the shorter sequences (n=2 and 4) form weak networks that are not able to maintain structural integrity due to the shearing-induced perturbation and, therefore, their network conductance drops to zero (c). (d) The distribution histograms of the numbers of connected nodes for H(AB)4and H(AB)12after shear flow. The H(AB)12sequence has node connectivity distribution peaks at higher values (∼5) than H(AB)4(∼2). Figure 4: Time evolution of the polymer network properties for the H(AB) n sequences. ( a ) Median number of ‘a’ beads per node as a measure of the aggregate size. ( b ) The total number of bridges as a measure of the connectivity. ( c ) The polymer network conductance as a measure of the degree of protein alignment. During both equilibration and shear flow, the median sizes of nodes do not vary a lot among all sequences ( a ), but longer copolymers have significantly more bridges ( b ). During shear flow, copolymers are stretched under shear flow and the cross-links are continuously broken and reformed until the steady state is reached for the simulated polymer properties in a – c . Although the network connectivity is not increased (in fact, it drops by a little due to shearing-induced perturbation) during shear flow ( b ), the network conductance for the long sequences ( n =8 and 12) are greatly enhanced due to the shearing-induced polymer alignment ( c ). The discontinuity between shear flow and tensile stretching periods in a – c is due to the stress relaxation simulation (results not reported here) in between the two periods. Interestingly, the shorter sequences ( n =2 and 4) form weak networks that are not able to maintain structural integrity due to the shearing-induced perturbation and, therefore, their network conductance drops to zero ( c ). ( d ) The distribution histograms of the numbers of connected nodes for H(AB) 4 and H(AB) 12 after shear flow. The H(AB) 12 sequence has node connectivity distribution peaks at higher values ( ∼ 5) than H(AB) 4 ( ∼ 2). Full size image To further understand the effect of shear flow on fibre formation, we introduce the measure of network conductance that characterizes the degree of anisotropic polymer alignment and network integrity (percolation) along the x axis (see Methods). Although the total number of bridges is not enhanced during shear flow ( Fig. 4b ), the network conductance is greatly increased during shear flow ( Fig. 4c ). This reveals the most important influence of shear flow in helping align the originally isotropic polymer chains and assemble them into anisotropic structures with good network connections. Interestingly, only the conductance of longer protein sequences ( n =8 and 12) are enhanced during shear flow, while the shorter ones drop to zero due to flow-induced disruption only along the x axis. This orientational effect, as a result of the shear flow, determines the critical polymer length ( n ≥8) beyond which silk formation becomes possible. A theoretical model based on the network percolation theory is used to explain such critical polymer length, as well as the optimal ‘A’–‘B’ domain ratio observed above (see Supplementary Discussion ). More importantly, shearing-induced polymer alignments need to overcome flow-induced network perturbations to sustain structural integrity along the x axis. Therefore, longer protein sequences are better candidates due to their pre-existing multiply connected network even before shear flow. Anisotropic polymer network conductance and fibre mechanics To understand the effect of polymer network microstructures on mechanical properties of the silk fibres, we performed tensile loading simulations on the network structures formed before and after shear flow ( Fig. 5a,b ). As expected from the enhanced number of bridges and conductance for longer sequences, the Young’s modulus is superior for longer protein chains both before and after shear flow. Specifically, the longest H(AB) 12 sequence leads to fibre formation after shear flow and exhibit the highest Young’s modulus of 3.5 MPa. Polymer networks formed before shear flow ( Fig. 5a ) are weak with softening behaviours at high tensile strains, while the ones formed after shear flow ( Fig. 5b ) exhibit stiffening behaviours. Interestingly, we found that after shear flow ( Fig. 5b ) the Young’s modulus of the network increases by about two times for longer sequences ( n =8 and 12), but drops to zero for shorter sequences ( n =2 and 4). The network microstructure evolution during tensile tests is shown in Fig. 5c for H(AB) 12 sequences, which exhibits three deformation steps: extension of individual polymer chains and bridges (soft hydrophilic ‘B’ domains forming amorphous phases) between clusters (stiff hydrophobic ‘A’ domains forming cross-linked β-sheet crystals), the escape and breakage of polymer chains from the cluster and sequential unfolding of polymer chains in the cluster. Our simulation results confirm the proposed deformation mechanism from the experimental tensile loading test of silk fibre accompanied by X-ray scattering [38] . 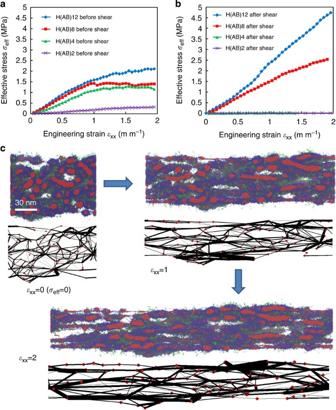Figure 5: Tensile mechanical tests of the H(AB)nsequences using the mesoscale model. (a,b) Stress–strain curves for mechanical tensile tests of polymer networks before and after shear flow. Before the shear flow, all networks are weak without stiffening at high tensile strains (low maximum stress), and it follows the trend that longer sequences are stronger with higher Young's modulus. After the shear flow, the network Young's modulus remains the same except that the Young's modulus for the two shorter sequences (n=2 and 4) drops to zero, and the longer sequences are stronger with much higher maximum stress and stiffening behaviour at high tensile strains. Note that due to the coarse-grained nature of the DPD model, the absolute stress values are approximate and we will focus on the relative values and comparisons among different protein sequences in a qualitative way. This factor, in addition to the presence of solvents in simulations, would also lead to simulated ultimate network strains much higher than that of common silk fibres (10%∼30%, ref.36.) Therefore, simulation predicted quantitative Young's modulus values are not to be compared with the later experimental tensile testing results. (c) Schematic of the H(AB)12network deformation process under various tensile strains. The red clusters (stiff cross-linked β-sheet crystals) slightly deform during stretching and maintain their structural integrity, while the blue bridges (soft amorphous regions) deform significantly or even break to release the applied stress. Figure 5: Tensile mechanical tests of the H(AB) n sequences using the mesoscale model. ( a , b ) Stress–strain curves for mechanical tensile tests of polymer networks before and after shear flow. Before the shear flow, all networks are weak without stiffening at high tensile strains (low maximum stress), and it follows the trend that longer sequences are stronger with higher Young's modulus. After the shear flow, the network Young's modulus remains the same except that the Young's modulus for the two shorter sequences ( n =2 and 4) drops to zero, and the longer sequences are stronger with much higher maximum stress and stiffening behaviour at high tensile strains. Note that due to the coarse-grained nature of the DPD model, the absolute stress values are approximate and we will focus on the relative values and comparisons among different protein sequences in a qualitative way. This factor, in addition to the presence of solvents in simulations, would also lead to simulated ultimate network strains much higher than that of common silk fibres (10% ∼ 30%, ref. 36 .) Therefore, simulation predicted quantitative Young's modulus values are not to be compared with the later experimental tensile testing results. ( c ) Schematic of the H(AB) 12 network deformation process under various tensile strains. The red clusters (stiff cross-linked β-sheet crystals) slightly deform during stretching and maintain their structural integrity, while the blue bridges (soft amorphous regions) deform significantly or even break to release the applied stress. Full size image In support of our modelling results, we carried out a series of experimental studies that focused on the H(AB) 12 sequences (see Supplementary Methods and Supplementary Fig. 5 ). SEM images of H(AB) 12 in aqueous solutions show fibre-like structures and nano-fibre (within the film) features for self-assembled H(AB) 12 polymers ( Supplementary Fig. 5a ), suggesting a high possibility of them forming silk fibres in a shear flow device. The original dried H(AB) 12 film Young's modulus was characterized using AFM nanoindentation. The resulting Young's modulus map and distribution show that the original H(AB) 12 films possess a Young’s modulus of only 20 ∼ 40 MPa ( Supplementary Fig. 5b ). Successful spinning of macroscopic fibres ( ∼ 1 cm long) using the H(AB) 12 sequence dissolved in two different solvents (aqueous LiBr solution and hexafluoroisopropanol (HFIP) with formic acid) is confirmed by both bright-field optical microscope and SEM images ( Fig. 6 ). The resulting concentrated silk solution was dialysed extensively against water to remove unnecessary LiBr ions (with a dilution factor of 1 to 2,000), which could be close to the natural spider silk-spinning condition (ionic environment with Na + and K + , ref. 30 ) and is consistent with the DPD modelling framework. The syringe needle fibre-spinning method is used here. As shown in Fig. 6a , H(AB) 12 polymers dissolved in HFIP can be spun into fibres that form bundles in the 2-propanol coagulation bath, consistent with our model predictions for longer chain polymers. The bundle delaminates and supercontracts after rehydrating by water, which results in individually separated fibres with relatively uniform diameters ( D ∼ 8 μm) under SEM ( Fig. 6b ). The hierarchical structure of the fibre bundle after 2-propanol treatment (dried without hydration) was probed in a series of SEM images ( Supplementary Fig. 6 ), showing the spherical H(AB) 12 protein aggregates as the fundamental building block of the fibre bundle, similar to our model-predicted morphology in Fig. 3d . In addition, H(AB) 12 polymers dissolved in aqueous LiBr solution form thinner individual fibres ( D ∼ 3 μm for dried fibres) without bundling ( Fig. 6c,d ). On the other hand, shorter sequences such as H(AB) 2 only form disordered films when dissolved in both solvents ( Supplementary Fig. 7 ), which is in good agreement with our model predictions about the effect of polymer chain length on fibre formation. 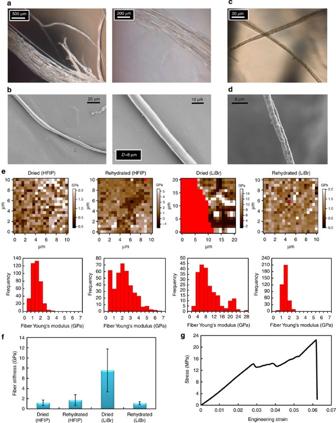Figure 6: Experimental validations for fibre spinning and mechanical properties. Syringe needle spinning of recombinant silk fibres with the H(AB)12polymer dissolved in HFIP: (a) bright-field microscopic images of spun fibres in bundle in the coagulation bath and (b) SEM images of the separated fibre after rehydration, showing a relatively uniform fibre diameter of∼8 μm. In addition, H(AB)12polymer dissolved in LiBr aqueous solution can also form thinner silk fibres without bundling: (c) bright-field microscopic images in the coagulation bath and (d) SEM images of the dried fibre showing a diameter of∼3 μm. Mechanical properties of syringe needle spun silk fibres using the H(AB)12sequence dissolved in two different solvents (HFIP and LiBr aqueous solution). The effect of hydration on fibre Young's modulus is studied by comparing air dried and rehydrated fibres. (e) The Young's modulus maps (top) and the corresponding Young's modulus distributions (bottom) of the four different types of fibres were obtained using the similar nanoindentation measurement as inSupplementary Fig. 5b. The red colour in the Young's modulus map indicates outliers with extremely high Young's modulus values. (f) Averaged fibre Young's modulus values over the distribution plots ine, showing standard deviations. (g) Representative stress-strain curve from mechanical tensile testing on various silk fibre samples, confirming high fibre robustness and Young's modulus. Figure 6: Experimental validations for fibre spinning and mechanical properties. Syringe needle spinning of recombinant silk fibres with the H(AB) 12 polymer dissolved in HFIP: ( a ) bright-field microscopic images of spun fibres in bundle in the coagulation bath and ( b ) SEM images of the separated fibre after rehydration, showing a relatively uniform fibre diameter of ∼ 8 μm. In addition, H(AB) 12 polymer dissolved in LiBr aqueous solution can also form thinner silk fibres without bundling: ( c ) bright-field microscopic images in the coagulation bath and ( d ) SEM images of the dried fibre showing a diameter of ∼ 3 μm. Mechanical properties of syringe needle spun silk fibres using the H(AB) 12 sequence dissolved in two different solvents (HFIP and LiBr aqueous solution). The effect of hydration on fibre Young's modulus is studied by comparing air dried and rehydrated fibres. ( e ) The Young's modulus maps (top) and the corresponding Young's modulus distributions (bottom) of the four different types of fibres were obtained using the similar nanoindentation measurement as in Supplementary Fig. 5b . The red colour in the Young's modulus map indicates outliers with extremely high Young's modulus values. ( f ) Averaged fibre Young's modulus values over the distribution plots in e , showing standard deviations. ( g ) Representative stress-strain curve from mechanical tensile testing on various silk fibre samples, confirming high fibre robustness and Young's modulus. Full size image The mechanical properties of four different types of spun fibres (with two solvent, and for air dried or rehydrated cases) were characterized using AFM nanoindentation ( Fig. 6e ). The rehydrated fibres will fill the purpose of testing the effect of hydration on fibre mechanics. Overall, the spun H(AB) 12 fibres exhibit a greatly enhanced Young's modulus modulus of 1 ∼ 8 GPa ( Fig. 6f ), with two orders of magnitude enhancement over the original dried films ( Supplementary Fig. 5 (b) ). More excitingly, the spun fibres here are very close to natural spider silk fibres with an initial Young's modulus of 3 ∼ 20 GPa, depending on spider species [36] , [39] . Mechanical tensile testing along the fibre axis also confirms their robustness with a tensile strength of ∼ 23 MPa, a Young’s modulus of ∼ 500 MPa and an ultimate strain of 6% ( Fig. 6g ). The fibre tensile testing results are not comparable with the nanoindentation results due to the fact that the tensile loading was introduced on fibre bundles (>100 μm in diameter) instead of individual fibres (<10 μm in diameter), for which individual fibre sliding along the pulling direction would diminish the ultimate fibre mechanical performance. These experimental findings agree very well with the model-predicted enhancement in the polymer network Young's modulus modulus after shear flow treatment ( Fig. 5 ), confirming that flow-focusing and shearing in the spinning process can indeed facilitate the assembly of silk fibres by aligning individual polymer chains. On the basis of the simulation results for the H(AB) n sequences, we summarize the correlation between various steady-state polymer network and mechanical properties with the number of repeated polymer units n in Fig. 7a . In general, all polymer networks and mechanical properties (aggregate size, network connectivity, network conductance and Young’s modulus) correlate well with the value of n , except that the network conductance and both mechanical properties remains zero for shorter chain lengths ( n =2 and 4) after shear flow due to destruction of the network along only the fibre axis. More importantly, we summarize the correlation between total number of bridges and conductance with the resulting Young’s modulus in Fig. 7b . The total number of bridges correlates well with the Young’s modulus before shear flow, as predicted by classical polymer theory, but cannot explain the zero Young’s modulus for shorter chains ( n =2 and 4) after shear flow ( Fig. 7b , top). This is because the total number of bridges does not represent the heterogeneity of the network connectivity and thus cannot capture the percolation of network. On the other hand, the network conductance not only explains the zero Young’s modulus for shorter chains ( n =2 and 4) after shear flow, but also exhibits perfect linear correlation with the Young’s modulus for all polymer chain lengths both before and after shear flow ( Fig. 7b , bottom) because it measures the contribution from the bridges to the anisotropic silk Young's modulus along the fibre axis. We can demonstrate the perfect correlation between the network conductance and the Young’s modulus by making an analogy between elastic spring network and resistance network (see Supplementary Discussion and Supplementary Fig. 8 ), extending the prediction of the classical polymer theory to heterogeneous fibres (recovering the limiting homogeneous case). As a result, we find that the network conductance instead of the total number of bridges is a good measure of network connectivity and thus is a key parameter for the predictive design of biological silk fibres, as demonstrated in Fig. 7b . 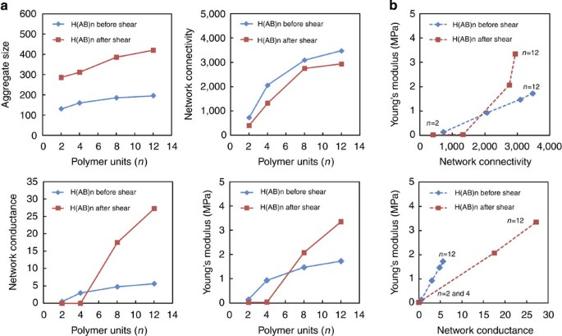Figure 7: Summary of modelling results and fibre design trends. (a) The effect of polymer chain length (measured by the number of repeated polymeric units,n) of the H(AB)nsequences on simulated steady-state polymer network properties, and the corresponding Young’s modulus before and after shear flow. All three polymer network properties correlate well with the value ofn, except that the network conductance remains zero for shorter chain length (n=2 and 4) after shear flow due to shearing-induced perturbations. The Young’s modulus also correlates well with the value ofn, except that, forn=2 and 4, the mechanical values remain zero after shear flow, as a result of discontinuous networks with zero conductance. (b) Correlations between total number of bridges and conductance of the H(AB)nsequences with simulated Young’s modulus. The total number of bridges correlates with the Young’s modulus before shear flow, but cannot explain the zero values for shorter chains (n=2 and 4) after shear flow. On the other hand, the network conductance correlates perfectly well with the Young’s modulus both before and after shear flow, representing an extension of the classical polymer theory to heterogeneous fibres (seeSupplementary Fig. 8). Figure 7: Summary of modelling results and fibre design trends. ( a ) The effect of polymer chain length (measured by the number of repeated polymeric units, n ) of the H(AB) n sequences on simulated steady-state polymer network properties, and the corresponding Young’s modulus before and after shear flow. All three polymer network properties correlate well with the value of n , except that the network conductance remains zero for shorter chain length ( n =2 and 4) after shear flow due to shearing-induced perturbations. The Young’s modulus also correlates well with the value of n , except that, for n =2 and 4, the mechanical values remain zero after shear flow, as a result of discontinuous networks with zero conductance. ( b ) Correlations between total number of bridges and conductance of the H(AB) n sequences with simulated Young’s modulus. The total number of bridges correlates with the Young’s modulus before shear flow, but cannot explain the zero values for shorter chains ( n =2 and 4) after shear flow. On the other hand, the network conductance correlates perfectly well with the Young’s modulus both before and after shear flow, representing an extension of the classical polymer theory to heterogeneous fibres (see Supplementary Fig. 8 ). Full size image In conclusion, we provide a generic design principle for general multiblock copolymers (A p B q ) n : (i) intermediate p : q ratio leads to balanced hydrophobicity, which is desirable to process homogeneous gels with well-connected polymer networks both before and during spinning, and (ii) large n value not only enhances network connectivity before spinning but is also necessary to retain network percolation against shear-induced disruption. Although longer protein sequences are preferred, the solubility of copolymers decreases as the length increases due to entropy reduction, which sets a limit on n to maintain solubility. Also, longer copolymer chains have slower dynamics, which could not be processed appropriately during the allowed processing time for shear flow spinning. To extend the simulation to much longer polymers approaching that of native silk proteins, a more time-efficient computational approach is in progress, for example, by modelling solvent molecules implicitly. We reveal that the anisotropic conductance of polymer networks (the alignment of bridges and percolation property) is more critical than the cross-linked β-sheet crystals and the total number of bridges for the ultimate mechanical properties of the silk fibre. Thus, we establish that network conductance is a proper measure of network connectivity and Young's modulus. Overall, this work systematically studies the sequence–structure–process–property relationships for producing artificial silk fibres using synthetic silk protein sequences and optimized shear-flow fibre-assembly protocol. In this work, we extended classical polymer theory, which describes only homogeneous polymer aggregates, with insights from a percolation network model that also is capable of describing heterogeneous polymer networks after spinning. The scalable models presented here, validated by experiments, can enable predictive designs of hierarchical materials with not only outstanding mechanical, but also promising transport properties (optical, electrical, thermal and others) by constructing network topologies and models that capture material structures and features at the molecular level. DPD simulation setup All DPD simulations are carried out using the massively parallelized LAMMPS package [40] . The simulations run in an elongated rectangular box (60 × 40 × 40 R c 3 , where R c =9.321 Å is the characteristic/physical length scale in the DPD model here) with a square cross-section and periodic boundary condition. The box length in the x axis (direction of flow) was chosen to be longer than a single extended chain, to avoid artifacts from boundary conditions. The concentration is fixed to 20% volume fraction of coarse-grained polymer beads (each representing three amino acids) in all the cases to match the experimental spinning condition. The total number of beads in a system is 288,000 for studying the HAB 3 , H(AB) 2 and HA 3 B systems. Note that when comparing among the H(AB) n ( n =2, 4, 8 and 12) systems, the simulation box size is increased to 120 × 80 × 40 R c 3 with a total number of 1,152,000 beads due to the longer polymer chains involved. For the starting structure, we grow peptides chains randomly with a fixed distance a (where a is the equilibrium bond distance in the chain) between beads in the simulation box, up to 20% of the volume fraction. We then fill the box with solvent beads until the number density of 3 is reached. After creating the initial random structure, we simulate the spinning process via several steps. All DPD simulations run under the NVE ensemble with a fixed time step of Δ t =0.03 τ , where τ =0.75 ns is the characteristic/physical time scale in the DPD model here. First, equilibration simulation is performed until a steady state is achieved, by tracking root-mean-square-deviation for 210,000 time steps. Second, a shear rate of is applied along the x axis (normal to the y axis) for 420,000 time steps to mimic the fibre-spinning process. The Lees–Edwards boundary conditions were applied to generate the shear flow [41] such that the same shear rate above was applied to all the materials in the system. Details on the DPD formalism and the parameterization procedure can be found in the Supplementary Methods . Equilibrations of self-assembled aggregates without and with shear flow were confirmed by the plateau in the time evolutions of the size of aggregates (or number of beads per node) and the number of bridges before shear (the equilibration period) and during the shear flow ( Figs 2 and 4 ), respectively. Another 100,000 time steps without shear were used to equilibrate the system after the shear flow, followed by the tensile simulations below. The aggregates that are enlarged due to shear flow will not break up after cessation of shear, although minor breakups were observed for aggregates composed of polymers of shorter chain length (data not shown). This implies that the simulated system after shear (with larger aggregates and better network connectivity) is kinetically (not thermodynamically) stable, compared with the thermodynamically stable system (with smaller aggregates and fewer network connections) before shear. The energy barrier for the transition from the sheared state to a lower energy state would be higher for longer polymers, possibility due to the entanglement (gelation) of longer chains, which prevents immediate aggregate breakups during the relatively short equilibration run. Polymer network analysis We define that two ‘a’ beads in the ‘A’ domain are connected if they are located within 0.94 R c , which is the averaged value of the first neighbour–neighbour distance 0.78 R c and the second neighbour–neighbour distance 1.10 R c . A cluster, that is, the aggregated β-sheet crystals (cross-linked via hydrogen bonds), is defined as the group of connected ‘a’ beads. The depth-first search algorithm is used to find the cluster distribution efficiently. Once cluster distribution is obtained, each isolated cluster is defined as a ‘node’ whose coordinate is defined as the centre of mass of ‘a’ beads in the cluster. Two nodes are defined to be connected with one ‘bridge’ if they are linked via the ‘B’ domain of at least one polymer chain. The number of connections between two nodes is defined as the multiplicity of the bridges, that is, the number of polymers through which they are linked. On the basis of the node connectivity, adjacency matrix is constructed that is used to generate the node–bridge diagrams. The conductance of the polymer network along the x axis is computed by drawing conceptual parallels with the resistance model of a typical electrical network [42] , in which one bridge possesses a conductance of 1 (that is, the no bridge case possesses zero conductance) and a voltage of 1 is applied between the left and the right boundaries. A similar study was reported recently on the structural network evolution of colloidal gels under shear flow using Brownian dynamics simulations [43] . Mechanical property modelling The mechanical property of the copolymer network before and after applying the shear flow is investigated using the standard tensile simulations along the x axis. The entire simulation box containing copolymers and the solvents is stretched in the x axis at a constant engineering strain rate of 7.5 × 10 −6 τ −1 , while the y and the z dimensions are adjusted simultaneously (with their aspect ratio fixed) to maintain the constant volume of the simulation box. The Young's modulus (Young’s modulus) of the network in the x axis, E x , can be obtained from the three-dimensional system using the equation: , where σ i ( i = x , , and z ) is the normal stress tensor value along the i axis, ɛ x is the strain along the x axis, and the Poisson’s ratio ν =0.5 for the constant volume constraint we enforced (incompressible). The effective stress can be then defined as σ eff = σ x − ν ( σ y + σ z ) and the linear-elastic region (for ɛ x ≤50%) of the stress–strain curve is used for determining E x . To remove the effect of solvents on E x , we corrected the value of E x by dividing it with the ratio between the volume of the entire simulation box and the effective volume occupied by the assembled copolymers. The DPD units for stress/pressure is k B T / R c 3 =1, which can be converted to the physical units of 5.11 MPa at 300 K. Note that the simulated system right after shear flow is already pre-stretched with σ eff >0 and therefore, a compressive simulation (using the same method as the tensile simulation, but with a negative strain rate of −5 × 10 −6 τ −1 ) is carried out first to relax the system and determine the stress-free configuration at which σ eff =0. The stress-free system, with a reduced box dimension along the x axis ( ∼ 70% of the original value), is then used as the new reference for the subsequent tensile simulation. Silk block copolymer biosynthesis and characterizations Synthetic or recombinant multiblock copolymer-like silk peptides and proteins (HAB 3 , HA 3 B and H(AB) n ( n =2, 4, 8 and 12) sequences) were cloned, expressed and purified according to the previously established procedure by Rabotyagova et al . [44] , [45] The purity of expressed proteins was verified by SDA–polyacrylamide gel electrophoresis (SDS–PAGE) electrophoresis followed by Colloidal Blue staining. Protein identity was confirmed by matrix-assisted laser desorption ionization mass spectrometry (Tufts Core Chemistry Facility, Boston, MA). SEM was used to assess morphological characterization of all spider silk block copolymers. The experiments were performed using a Zeiss 55Ultra System (Harvard University Center for Nanoscale Systems, Cambridge, MA). Each sample was sputter-coated with platinum with a HAR024 sputter coater and mounted onto a sample holder with conductive tape. Lyophilized peptides were dissolved in water to a final concentration of 1 mg ml −1 and dried on a silicon chip in a closed container at room temperature. Images were taken using InLense and SE2 detectors at 1 keV. Sample dried films ∼ 10 μm in thickness were cast onto CaF 2 substrate for the FTIR spectroscopy measurements. FTIR was carried out on a Jasco FT/IR-6200 spectrometer with a TGS detector. The absorbance spectra were obtained by averaging 128 scans with a resolution of 4.0 cm −1 . The background spectra were collected under the same conditions and subtracted from the scan for each sample. We then carried out Fourier self-deconvolution over the amide I peaks on the resulting FTIR spectra, using Opus 5.0 software with Lorentzian peak profile (half-bandwidth of 25 cm −1 and a noise reduction factor of 0.3). This renders individual spectrum, which was used to obtain the composition (in percentage) of different protein secondary-structure contents by integrating the area of each deconvoluted curve, and then normalizing to the total area of the amide I peak. FTIR spectra and the corresponding Fourier self-deconvolution data for the H(AB) 2 sequence and the H(AB) 12 sequence before and after spun are shown in Supplementary Fig. 9 . AFM imaging and force spectroscopy measurements were performed on an Asylum Research MFP-3D-Bio AFM (Asylum Research, an Oxford Instruments Company, Santa Barbara, CA). For imaging in fluids, 80 μl sample of 1% w/v was deposited as a drop on a silicon substrate and imaged. IgorPro 6.22A image analysis software was used to determine the heights of observed structures. The root-mean-square and the arithmetic average height ( R a) were determined using software to find differences between roughnesses of samples. Force curves were obtained with AFM in the contact mode. All imaging was performed in contact mode using Olympus silicon probes on a silicon surface. Cantilever specifications are the following: 160 μm in length, 40 μm in width, with a resonant frequency of 300±50 kHz. Syringe spinning of silk fibres and characterization Syringe fibre spinning was carried out following the protocol in previous work [46] using 15% w/v recombinant silk protein solutions, H(AB) 2 and H(AB) 12 , synthesized in this work. The experimental setup is shown in Supplementary Fig. 10 , with two different solvents (95% HFIP with 5% formic acid, or 9 M LiBr aqueous solution after 1-h dialysis against water) being used for dissolving the proteins to fine-tune their aggregation. The extensive dialysis (100 ml solution against 2 l water) removes unnecessary ions. In brief, the protein solutions are extruded at a speed of 15 μl min −1 through a stainless-steel syringe needle (22 G, 127 micron, Hamilton) into 90% 2-propanol coagulation bath to form fibres. The spinning mimics aspects of native silk processing in a tunable manner via hydrodynamic flow focusing and shearing. After the fibres were formed (only with H(AB) 12 ) and air dried, we rehydrated some of them by immersing them into water to study the hydration effect on fibre mechanical properties. SEM images were taken on each fibre sample with the same parameters mentioned earlier except that the operating voltage was enhanced to 5 keV with an InLense detector. AFM nanoindentations of the original dried H(AB) 12 films and the spun H(AB) 12 fibres were carried out using the same AFM device mentioned earlier. Local Young's modulus (Young’s modulus) of the film was calculated using the force versus indentation depth curve ( Supplementary Fig. 11 ) and based on detailed procedures and equations in the work by Spedden and Staii [47] . The Young's modulus map and distribution were obtained by scanning a squared region (20 × 20 μs 2 ) on each sample and collecting various local Young's modulus values on a much smaller subregion (2 × 2 μs 2 ). The indentations on four different types of H(AB) 12 fibres (dissolved in two solvents, dried or rehydrated) were carried out using an AC160TS-R3 cantilever (spring constant 26 N m −1 ) on a 10 × 10 μs 2 squared region. Tensile measurements of spun fibres were performed on an Instron microtester (Instron, Norwood, MA) with a 5 N load cell. Samples were stuck to a custom frame to prevent them from breaking prematurely. Once the samples were loaded, the frames were removed and the fibres were pulled at 0.01 s −1 strain rate until failure. Force data were collected and normalized to stress values on the basis of respective diameter measurements. Fibre diameters were determined using light microscopy under × 20 magnification. How to cite this article: Lin, S. et al . Predictive modelling-based design and experiments for synthesis and spinning of bioinspired silk fibres. Nat. Commun . 6:6892 doi: 10.1038/ncomms7892 (2015).